Weakening of the stratospheric polar vortex by Arctic sea-ice loss Successive cold winters of severely low temperatures in recent years have had critical social and economic impacts on the mid-latitude continents in the Northern Hemisphere. Although these cold winters are thought to be partly driven by dramatic losses of Arctic sea-ice, the mechanism that links sea-ice loss to cold winters remains a subject of debate. Here, by conducting observational analyses and model experiments, we show how Arctic sea-ice loss and cold winters in extra-polar regions are dynamically connected through the polar stratosphere. We find that decreased sea-ice cover during early winter months (November–December), especially over the Barents–Kara seas, enhances the upward propagation of planetary-scale waves with wavenumbers of 1 and 2, subsequently weakening the stratospheric polar vortex in mid-winter (January–February). The weakened polar vortex preferentially induces a negative phase of Arctic Oscillation at the surface, resulting in low temperatures in mid-latitudes. Over the past two decades, the Arctic Ocean has warmed significantly in conjunction with conspicuous increase in global surface air temperature (SAT) and rapid decline of Arctic sea-ice [1] , [2] . A growing number of studies have found pronounced changes in atmospheric circulation due to Arctic sea-ice loss, including changes in the tropospheric jet stream that may lead to cold extremes over Eurasia and North America [3] , [4] , [5] , [6] , [7] . However, because the occurrence of major sea-ice losses has been relatively recent, a robust connection between Arctic sea-ice and atmospheric circulation has not been well-established, and the underlying mechanism(s) responsible for these processes are not yet fully understood [8] , [9] . For example, through the analysis of re-analysis data and climate model outputs, a number of studies have suggested that Arctic sea-ice loss has the potential to force the Arctic Oscillation (AO) into its negative phase [10] , [11] , [12] . In contrast, other recent studies have emphasized the impact of planetary-scale wave pattern over the Eurasian continent that emanates from the Barents–Kara (B–K) seas [4] , [13] , [14] . Apparently, this pattern appears to be zonally asymmetric and different from a typical pattern of the AO [15] . Efforts have also been made to relate the recent changes in cryospheric conditions such as Eurasian snow cover and Arctic sea-ice cover to the variability of the stratospheric polar vortex [16] , [17] , [18] . It is documented that the variability of the stratospheric polar vortex has increased in recent years. For instance, whereas the sudden weakening of the stratospheric polar vortex, known as a major Sudden Stratospheric Warming (SSW) event, occurred relatively infrequently during the 1990s according to the World Meteorological Organization (WMO) definition of SSW [19] , it has occurred almost every year since 2000 (ref. 20 ). SSW events are often followed by a negative phase of the AO at the surface with a time lag of 1 or 2 months [21] , [22] , [23] . This indicates that understanding possible contributors to recent stratospheric variability, which may include cryospheric changes [24] , is critical for the better understanding of the surface climate variability in the recent past. A systematic study that considers both bottom-up and top-down processes occurring within the cryosphere, troposphere and stratosphere is therefore crucial for elucidating how Arctic sea-ice interacts with atmospheric circulation and thereby causes extreme surface weather events. In this study, a time-lagged stratospheric response to Arctic sea-ice loss is examined via composite analyses that utilize both European Center for Medium-Range Weather Forecasts (ECMWF) Re-Analysis Interim (ERA-Interim) data [25] and climate model sensitivity experiments. This synthetic analysis reveals that polar stratospheric variability is partly controlled by marked losses of Arctic sea-ice, especially over the B–K seas. Sea-ice-polar vortex relationship from data analysis Arctic sea-ice losses in recent decades have been widely documented [26] . Our particular interest lies in sea-ice conditions during the early winter period (November–December) due to the potential impact of such conditions on mid-winter weather and climate patterns. During this season of recent years, the B–K seas have lost significant volumes of sea-ice while exhibiting pronounced interannual variations ( Fig. 1a,b ; ref. 15 ). A large amount of air–sea heat exchange is also observed during the years of anomalously low sea-ice concentration (SIC) over the B–K seas partly due to the occurrence of increased Atlantic warm water intrusion in recent years [27] . 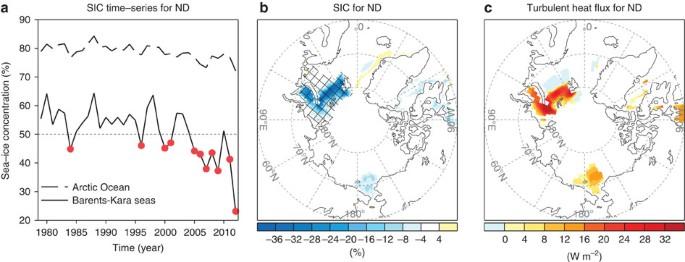Figure 1: SIC variability over the B–K seas during the early winter season. (a) An area-averaged time-series of SIC for the entire area of the Arctic Ocean (dashed) and B–K seas (solid) during the early winter for the period 1979–2012. The area of the B–K seas is indicated by hatched region inb. Years during which the area-averaged SIC <50% over the B–K seas are indicated by red dots (11 sample years). The composite mean anomaly of (b) SIC (%) and (c) surface turbulent heat flux (W m−2; the sum of sensible and latent heat flux) for the years indicated by the red dots ina. Anomaly is defined as a departure from climatology data for the period 1979–2012. Figure 1: SIC variability over the B–K seas during the early winter season. ( a ) An area-averaged time-series of SIC for the entire area of the Arctic Ocean (dashed) and B–K seas (solid) during the early winter for the period 1979–2012. The area of the B–K seas is indicated by hatched region in b . Years during which the area-averaged SIC <50% over the B–K seas are indicated by red dots (11 sample years). The composite mean anomaly of ( b ) SIC (%) and ( c ) surface turbulent heat flux (W m −2 ; the sum of sensible and latent heat flux) for the years indicated by the red dots in a . Anomaly is defined as a departure from climatology data for the period 1979–2012. Full size image In conjunction with anomalously low SIC over the B–K seas, the composite SAT anomaly (see Methods) has exhibited a “warm Arctic and cold continent” pattern [15] , [28] , with significant warming of up to 4 °C over the Arctic Ocean and a cooling of 2 °C over Siberia ( Fig. 2a ). The warm temperatures over the Arctic Ocean correspond closely with regions that experience major sea-ice losses during the early winter months ( Fig. 1b ). This pattern demonstrates the critical role of turbulent heat fluxes resulting from increases in the area of open water [27] , as such warm water causes heat fluxes to release extensive levels of heat into the atmosphere during this period of the year ( Fig. 1c ). Large-scale circulation changes also occur within the mid-troposphere, resulting in the development of a positive height anomaly over the B–K seas ( Fig. 2b ). The height anomaly follows a wave-like pattern, that is, a negative anomaly develops over Western Europe, a positive anomaly forms over the B–K seas, and a negative anomaly forms over Siberia. Note that the local warm and cold centres of SAT anomalies shown in Fig. 2a largely collocate with the wave-like pattern shown in Fig. 2b . This coincidence suggests that Siberian cooling may be attributable to the development of a planetary-scale wave train that is induced by sea-ice loss in the B–K seas. 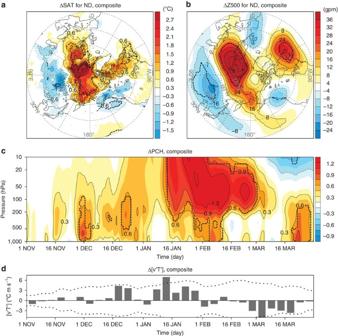Figure 2: Composite mean differences during the years of reduced Arctic sea-ice. Composite mean differences from climatology data with respect to (a) surface air temperature, (b) the geopotential height anomaly at 500 hPa for the early winter, (c) the subseasonal evolution of the PCH as a function of pressure and (d) 5-day averaged composite poleward heat flux anomalies at 100 hPa from ERA-Interim data. Inaandb, contour intervals are 0.3 °C and 4 m, respectively. Inc, the contour interval is 0.3. Values that are statistically significant at the 95% confidence level are enclosed by a dotted line (see Methods). Figure 2: Composite mean differences during the years of reduced Arctic sea-ice. Composite mean differences from climatology data with respect to ( a ) surface air temperature, ( b ) the geopotential height anomaly at 500 hPa for the early winter, ( c ) the subseasonal evolution of the PCH as a function of pressure and ( d ) 5-day averaged composite poleward heat flux anomalies at 100 hPa from ERA-Interim data. In a and b , contour intervals are 0.3 °C and 4 m, respectively. In c , the contour interval is 0.3. Values that are statistically significant at the 95% confidence level are enclosed by a dotted line (see Methods). Full size image Polar vortex variability can be readily assessed using the polar cap height (PCH) anomaly, which is obtained from the area-averaged geopotential height anomaly over the area north of 65 ° N, normalized by the standard deviation for each of the standard 26 pressure levels [29] . By definition, the existence of a positive PCH anomaly corresponds to a weakened polar vortex and can be related to the negative phase of the Northern Annular Mode. The surface PCH anomaly is linearly correlated with the AO index [29] . To identify the linkage between the sea-ice and the stratospheric polar vortex variability, a composite analysis is conducted as a function of time and pressure ( Fig. 2c ). Figure 2c shows the seasonal evolution of the composite PCH anomaly for the years of anomalously low SIC over the B–K seas. The positive PCH anomaly dominates for the majority of winters, indicating a weakening of the polar vortex. However, the behaviour of the polar vortex during early winter differs from that in mid-winter (January–February). During early winter, the positive PCH anomaly remains largely confined to the troposphere and tends to be relatively weaker in magnitude than during mid-winter. The pattern depicted in Fig. 2b , which is asymmetric in the zonal direction, contributes to the development of a positive PCH tropospheric anomaly during the early winter months. In contrast, beginning in early January, a positive PCH anomaly appears in the upper stratosphere that descends thereafter, indicating the possible dynamic coupling between the stratosphere and troposphere. In the later section, we will show that this weakening of the stratospheric polar vortex in early January can be explained by the increased poleward heat flux anomalies at 100 hPa ( Fig. 2d ), which is the indicator of the vertical flux of wave activity from the troposphere. Modelling evidence The statistical analysis described above suggests that the development of a weakened mid-winter polar vortex in recent years may be attributed to the occurrence of sea-ice loss in the B–K seas. However, the robustness of the suggested relationship must be tested further as the analyzed relationships may have resulted due to chance given the small number of years used in the composite (11 years, indicated by red dots in Fig. 1a ). To support our findings, climate model experiments were performed using the Community Atmospheric Model Version 5 (CAM5), which is a newly developed, state-of-the-art climate model [30] , [31] . Two experiments, that is, control and sea-ice perturbed runs, were prepared (see Methods). They only differ in surface boundary conditions over the Arctic Ocean. Each experiment was composed of 40 independent runs of varying initial conditions to estimate ensemble-mean model responses. The modelled atmospheric response to sea-ice loss over the B–K seas is then defined as the difference between the ensemble mean of the perturbed runs and that of the control runs. For further details, see the Methods section. The modelled response successfully reproduces the overall response of the SAT and mid-tropospheric circulation to the anomalously low SIC over the B–K seas (compare Fig. 2a,b , and Fig. 3a,b ). In particular, similarities in the mid-tropospheric height anomalies over the Eurasian continent confirm that sea-ice loss over the B–K seas induces a planetary-scale wave train and contributes to Eurasian surface cooling. However, differences are also found between the modelled responses and composite anomalies especially over North America ( Fig. 3a,b ). These differences are likely attributable to the fact that the surface boundary condition in the model experiments is fixed everywhere except for the Arctic Ocean which is not the case in the composite analysis. 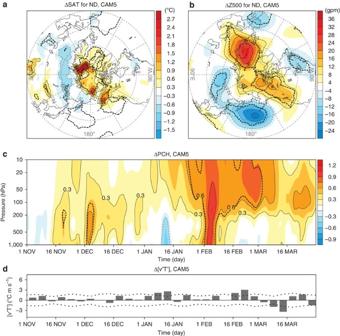Figure 3: Model ensemble-mean responses for the reduced Arctic sea-ice condition. Model ensemble-mean responses to the reduced SIC over B–K seas for (a) surface air temperature, (b) the geopotential height anomaly at 500 hPa for the early winter, (c) the subseasonal evolution of the PCH as a function of pressure and (d) 5-day averaged poleward heat flux anomalies at 100 hPa. Inaandb, contour intervals are 0.3 °C and 4 m, respectively. Inc, the contour interval is 0.3. Values that are statistically significant at the 95% confidence level are displayed by a dotted line (see Methods). Figure 3: Model ensemble-mean responses for the reduced Arctic sea-ice condition. Model ensemble-mean responses to the reduced SIC over B–K seas for ( a ) surface air temperature, ( b ) the geopotential height anomaly at 500 hPa for the early winter, ( c ) the subseasonal evolution of the PCH as a function of pressure and ( d ) 5-day averaged poleward heat flux anomalies at 100 hPa. In a and b , contour intervals are 0.3 °C and 4 m, respectively. In c , the contour interval is 0.3. Values that are statistically significant at the 95% confidence level are displayed by a dotted line (see Methods). Full size image In spite of this regional discrepancy, the modelled response captures a significant weakening of mid-winter polar vortex in the stratosphere ( Fig. 3c ) as in composite analysis ( Fig. 2c ). More importantly, the downward coupling between the stratosphere and troposphere occurring in late January and early February is effectively reproduced. The resulting tropospheric circulation anomaly then favors cold surface temperatures over Northern Hemisphere continents in late winter (January–March) ( Supplementary Fig. 1 ). Identical model experiments were also performed using CAM3, the previous version of CAM5 ( Supplementary Fig. 2 ). Despite significant differences in model physics and mean biases [31] , CAM3 experiments show essentially the same results to the CAM5 experiments. Although this consistency suggests that the modelling results may not be sensitive to the model physics and bias, further experiments using different models are needed to increase the robustness of our findings. Given the successful simulation of sea-ice-polar vortex relationships ( Fig. 3c ), it is worthwhile to examine whether noticeable differences in stratospheric variability exist between the two model experiments. Specifically, we count SSW events simulated by the control and perturbed runs. A widely used definition of SSW event, zonal mean zonal wind reversal at 60 ° N and 10 hPa, is employed here [32] . Out of the 40 ensemble members of the control and perturbed experiments, a total of 17 and 25 SSW events, or 0.35 and 0.64 events per year, were identified, respectively. This result is consistent with the more frequent occurrence of SSW events during the years exhibiting lower SIC over the B–K seas in the re-analysis data. The consistency was also found in the overall polar vortex variability, which was quantified from the frequency distribution of zonal mean zonal wind at 60 ° N at 10 hPa. Re-analysis data shows a slight increase in the frequency of weakened zonal winds during the years with low SIC ( Fig. 4a ), although insufficient sample size introduces uncertainty. Model experiments produce essentially the same results to the composite analysis with more visible frequency shifts toward the weaker winds ( Fig. 4b ). These results suggest that sea-ice loss over the B–K seas generally induces more frequent occurrence of weak vortex events. 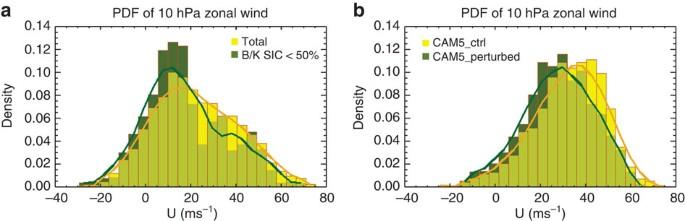Figure 4: Histogram summary of stratospheric variability. (a) The normalized frequency distribution of daily zonal mean zonal wind at 60°N at 10 hPa during the late winter for the period 1979–2012 (yellow) and for 11 years exhibiting SIC levels over the B–K seas that are <50% during early winter (green). (b) Same withaexcept for the model control experiment (yellow) and sea-ice perturbed experiment (green). In both figures, the solid line indicates a five-point histogram value average. Note that the two distributions in bothaandboverlap each other significantly. The overlapped region is visualized by different colour (light green). Figure 4: Histogram summary of stratospheric variability. ( a ) The normalized frequency distribution of daily zonal mean zonal wind at 60 ° N at 10 hPa during the late winter for the period 1979–2012 (yellow) and for 11 years exhibiting SIC levels over the B–K seas that are <50% during early winter (green). ( b ) Same with a except for the model control experiment (yellow) and sea-ice perturbed experiment (green). In both figures, the solid line indicates a five-point histogram value average. Note that the two distributions in both a and b overlap each other significantly. The overlapped region is visualized by different colour (light green). Full size image Upward wave propagation excited by Arctic sea-ice loss Based on the evidence derived from the statistical analysis of the observation-based dataset and numerical modelling results, a physical mechanism that explains the effect of Arctic sea-ice loss on the stratospheric polar vortex was investigated. We hypothesized that the positive stratospheric PCH anomaly is driven by Arctic sea-ice loss primarily through the vertical flux of wave activity from the troposphere. To test this hypothesis, we calculated the zonal-mean eddy heat flux, [v′T′], at 100 hPa averaged between 45°N and 75°N from both re-analysis and the model datasets [33] . Here, v is the meridional wind and T is the temperature at 100 hPa. The bracket and prime denote the zonal mean and the deviation from the zonal mean, respectively. This quantity has been widely used to quantify the intensity of vertically propagating wave activity. The composite [v′T′] anomaly using the re-analysis is shown in Fig. 2d and the ensemble-mean response of [v′T′] obtained by the model experiments is shown in Fig. 3d . Both demonstrate an emergence and gradual increase of vertical wave activity preceding the occurrence of the positive stratospheric PCH anomaly [33] . Notable wave activity begins in early winter from the lower troposphere and then extends to the stratosphere by the mid-winter months, accompanied by a dramatic increase in magnitude. This time evolution suggests that sea-ice reductions enhance vertical wave activity, which in turn produces a positive PCH anomaly or weak vortex in the stratosphere. Further analyses reveal that the tropospheric wave disturbance shown in Fig. 2b ( Fig. 3b for the model response) is the main driver of the enhanced vertical wave propagation during the early winter season. According to the quasi-geostrophic linear dynamics, vertically propagating waves should have zonal disturbances that are tilted westward with heights [34] . This westward tilting is observed in a wide range of waves ranging from synoptic to planetary scales. However, it is well-recognized that wavenumber 1 and 2 disturbances are the predominant waves that propagate into the winter stratosphere and subsequently weakening the polar vortex [34] . To examine the horizontal and vertical structures of sea-ice-induced planetary-scale waves that propagate into the stratosphere, the wave disturbance patterns depicted in Fig. 2b ( Fig. 3b for model response) are decomposed by wavenumber using a Fourier transformation along the latitude circle. 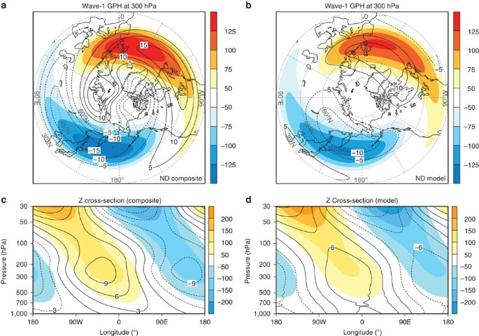Figure 5: Wavenumber 1 disturbance linked to Arctic sea-ice loss. (a) The zonal wavenumber 1 component of geopotential height at 300 hPa derived from ERA-Interim data. The composite anomaly (contour) from the selected years of reduced Arctic sea-ice levels (red dots inFig. 1a) is compared with the long-term climatology data (shading). (b) Same asaexcept for the model ensemble response (contour) and model climatology for the control simulation (shading). Contour and shading intervals are 5 m and 25 m, respectively. (c) and (d): Same asaandbwith the exception of the longitude-pressure section averaged over 45°N–75°N. Contour and shading intervals are 3 m and 50 m, respectively. Figure 5a presents the zonal wavenumber 1 component for the geopotential height field at 300 hPa. The zonal and vertical structure averaged over 45°N-75°N is also provided for the zonal wavenumber 1 component ( Fig. 5c ). The composite anomaly for the years with reduced sea-ice (contour) is compared with the long-term climatology value (shading). Similarly, the ensemble-mean response of the geopotential height field is compared with the control experiment mean ( Fig. 5b,d ). From these figures, the zonal and vertical structures of the zonal wavenumber 1 anomalies are approximately in phase with the long-term climatology for both the composite analysis and model simulations. Because wave energy is proportional to the square of wave amplitude, the wave that is in phase with climatological wave constructively interferes with it. This constructive interference also occurs in zonal wavenumber 2 at a weaker magnitude. Figure 5: Wavenumber 1 disturbance linked to Arctic sea-ice loss. ( a ) The zonal wavenumber 1 component of geopotential height at 300 hPa derived from ERA-Interim data. The composite anomaly (contour) from the selected years of reduced Arctic sea-ice levels (red dots in Fig. 1a ) is compared with the long-term climatology data (shading). ( b ) Same as a except for the model ensemble response (contour) and model climatology for the control simulation (shading). Contour and shading intervals are 5 m and 25 m, respectively. ( c ) and ( d ): Same as a and b with the exception of the longitude-pressure section averaged over 45°N–75°N. Contour and shading intervals are 3 m and 50 m, respectively. Full size image In the Arctic Ocean, the model response and composite analysis show notable differences in wavenumber 1 component. However, the vertical wave activity that controls the stratosphere is not sensitive to the circulation anomaly over the Arctic Ocean, where the climatological stationary wave is almost absent. Note that the vertical wave activity is, instead, determined by the eddy heat flux anomaly in mid-latitudes [33] . According to recent studies [35] , [36] , [37] , the linear interference of wavenumbers 1 and 2 largely determines the vertical wave activity of planetary-scale waves (see also Supplementary Fig. 3 ). Therefore, the result shown in Fig. 5 suggests that Arctic sea-ice anomalies tend to enhance vertically propagating planetary-scale waves by constructively interfering with climatological planetary-scale waves, which likely weakens the polar vortex. Upward wave propagation from the troposphere to the stratosphere has also been examined in the context of blocking highs in the troposphere. It has been argued that the occurrence of blocking at particular geographical locations, such as the B–K seas and Ural Mountain regions, can cause vertically propagating planetary-scale waves; therefore, the occurrence of blocking can be regarded as a tropospheric precursor to the stratospheric polar vortex weakening [36] , [38] , [39] . The present study supports this idea. Despite the regional differences, both the re-analysis and modelling datasets demonstrate that regional blocking near the B–K seas tends to occur more frequently and persist for much longer periods in low sea-ice conditions over the B–K seas ( Supplementary Fig. 4 ). This finding provides further evidence of Arctic sea-ice-related stratospheric changes. Through a combination of observation-based data analysis and climate model experiments, we provide corroborative evidence for the notion that Arctic sea-ice loss over the B–K seas plays an important role in weakening the stratospheric polar vortex. Regional sea-ice reductions over the B–K seas cause not only in situ surface warming but also significant upper-level responses that exhibit positive geopotential height anomalies over Eastern Europe and negative anomalies from East Asia to the Eastern Pacific along the wave-guide of the tropospheric westerly jet. This anomaly pattern projects heavily into the climatological wave, intensifying the vertical propagation of planetary-scale wave into the stratosphere and, in turn, weakening the stratospheric polar vortex. Therefore, planetary-scale wave generation by sea-ice losses and its upward propagation during early winter months underline the link between surface climate variability and polar stratospheric variability. The weakened stratospheric polar vortex is often followed by a negative phase of the AO at the surface [21] , [22] , [23] , favoring cold surface temperatures across Northern Hemisphere continents during the late winter months ( Supplementary Fig. 1 ). Several physical mechanisms for this downward coupling have been proposed. They include the balanced response of the troposphere to stratospheric potential vorticity anomalies and wave-driven changes in the meridional circulation [40] , [41] . It is also suggested that the tropospheric response involves changes in the synoptic eddies [42] , [43] . However, it has been difficult to isolate the key process, and the detailed nonlinear processes involved are still under investigation [21] . As a final remark, we note that Arctic sea-ice loss represents only one of the possible factors that can affect the stratospheric polar vortex. Other factors reported in previous works include Eurasian snow cover, the Quasi Biannual Oscillation, the El-Niño and Southern Oscillation and solar activity [24] , [44] , [45] . Systematic consideration of these factors would extend our understanding of climate variability, possibly leading to the improved seasonal forecast [46] . Nonetheless, the relative contributions of each factor have not been systematically examined. As these factors may be interrelated, they may not control the stratospheric polar vortex independently. These issues must be examined further in future works. Composite analysis SIC and Sea Surface Temperature (SST) are obtained from Hadley Centre Sea-Ice and SST data [47] . Eleven of the 34 years (1979–2012) during which the averaged SIC over the B–K seas shows an anomalously low fraction (<50%; red dots in Fig. 1a ) were selected for the composite analysis. Various meteorological fields including surface fluxes were obtained from ERA-Interim [25] and analyzed at a spatial resolution of 1.5 by 1.5 degrees. Surface turbulent heat fluxes in Fig. 1c were computed by combining sensible and latent heat fluxes, which are obtained from the ERA-Interim data. Model configuration and experimental design The CAM5 model was configured by a finite volume dynamical core with a horizontal resolution of 2.5° (longitude) by 1.9° (latitude) and 30 vertical levels extending to 3 hPa (~40 km). A common challenge faced in the process of Arctic climate simulation is the excessive wintertime low-level cloud in the model under extremely cold and dry conditions [48] , [49] . To reduce this bias, the model experiments in this study applied a modified formula for calculating fractions of low-level stratiform clouds (where air pressure levels ⩾ 750 hPa). A detailed description of the formula is provided in ref. 48 . Two sets of experiments were performed: that is, control and perturbed runs. The control experiment was conducted with a seasonal cycle of SIC and SST based on the climatology of the Hadley Centre SIC and SST for the period 1979–2012 (ref. 47 ). For the perturbed experiment, we introduced the composite seasonal cycle of SIC and SST to the Arctic Ocean during the years of reduced sea-ice, as indicated in Fig. 1a ( Supplementary Fig. 5 ). In this study, the Arctic Ocean is defined as the collection of grid points in which the SIC value is >15% within the Arctic Circle (north of 65°N) at least once during the period 1979–2012. For the regions outside of the Arctic Ocean, the same climatological SST condition that was used for the control simulation was applied for the perturbed runs. To obtain reliable model responses to the imposed sea-ice losses, both control and perturbed runs were conducted with 40 ensemble members by slightly varying atmospheric initial conditions. Each integration started on 1 April and terminated on 31 March, marking one full year of integration. The modelled atmospheric response is then defined as the ensemble-mean difference generated by subtracting the ensemble-mean values of the perturbed runs from those of the control runs. Statistical significance The statistical significance of the composite mean difference and model ensemble-mean difference shown in Figs 2 and 3 was determined by following a bootstrap resampling procedure by random sampling with the replacement of 10,000 samples. Because we applied the statistical test for each spatial grid point, we did not account the persistence in the time domain. Therefore, the area of statistical significance shown in Figs 2c and 3c (enclosed by the dotted line) may be an underestimated value. How to cite this article: Kim, B.-M. et al. Weakening of the stratospheric polar vortex by Arctic sea-ice loss. Nat. Commun. 5:4646 doi: 10.1038/ncomms5646 (2014).